TCF12is mutated in anaplastic oligodendroglioma Anaplastic oligodendroglioma (AO) are rare primary brain tumours that are generally incurable, with heterogeneous prognosis and few treatment targets identified. Most oligodendrogliomas have chromosomes 1p/19q co-deletion and an IDH mutation. Here we analysed 51 AO by whole-exome sequencing, identifying previously reported frequent somatic mutations in CIC and FUBP1 . We also identified recurrent mutations in TCF12 and in an additional series of 83 AO. Overall, 7.5% of AO are mutated for TCF12 , which encodes an oligodendrocyte-related transcription factor. Eighty percent of TCF12 mutations identified were in either the bHLH domain, which is important for TCF12 function as a transcription factor, or were frameshift mutations leading to TCF12 truncated for this domain. We show that these mutations compromise TCF12 transcriptional activity and are associated with a more aggressive tumour type. Our analysis provides further insights into the unique and shared pathways driving AO. Anaplastic oligodendrogliomas (AO; World Health Organization grade III oligodendrogliomas) are rare primary malignant brain tumours with a highly variable overall prognosis. The emblematic molecular alteration in oligodendrogliomas is 1p/19q co-deletion, which is associated with a better prognosis and response to early chemotherapy with procarbazine, lomustine and vincristine [1] , [2] , [3] . Recent high-throughput sequencing approaches have identified IDH ( IDH1 and IDH2 ), CIC , FUBP1 and TERT promoter mutations in oligodendroglioma (75, 50, 10 and 75%, respectively) [2] , [4] , [5] , IDH mutation status typically being associated with a better clinical outcome [6] . Identifying additional driver genes and altered pathways in oligodendroglioma offers the prospect of developing more effective therapies and biomarkers to predict individual patient outcome. Here we perform whole-exome and transcriptome sequencing of AO to search for additional tumour driver mutations and pathways disrupted. In addition to previously reported recurrently mutated genes, we report the identification of somatic mutations in TCF12 in AO. These mutations compromise TCF12 transcriptional activity and confer a more aggressive AO phenotype. In accordance with conventional clinical practice, we considered three molecular subtypes for our analyses: (i) IDH -mutated 1p/19q co-deleted ( IDH mut-codel); (ii) IDH -mutated 1p/19q non-co-deleted ( IDH mut-non-codel) and (iii) IDH -wild type ( IDH wt) [7] . Assignment of IDH -mutated (defined by IDH1 R132 or IDH2 R172 mutations), 1p/19q and TERT promoter mutation (defined by C228T or C250T) status in tumours was determined using conventional sequencing and single-nucleotide polymorphism (SNP) array methods. Mutational landscape We performed whole-exome sequencing of 51 AO tumours ( Supplementary Data 1 ) and matched germline DNA, targeting 318,362 exons from 18,901 genes. The mean sequencing coverage across targeted bases was 57 × , with 80% of target bases above 20 × coverage ( Supplementary Fig. 1 ). We identified a total of 4,733 mutations (with a mean of 37 non-silent mutations per sample) equating to a mean somatic mutation rate of 1.62 mutations per megabase (Mb) ( Fig. 1 ). Although the tumours of two patients (3,063 and 3,149) had high rates of mutation (9.1 and 12.4, respectively), this was not reflective of tumour site (both frontal lesions as were 68% of the whole series) or treatment. Excluding these two cases the mean rate of non-silent mutations per tumour was 33±14, which is similar to the number found in most common adult brain tumours. The mutation spectrum in AO tumours was characterized by a predominance of C>T transitions, as observed in most solid cancers ( Fig. 1 ) [8] , [9] . While few of the tumours were IDHwt , these did not harbour a significantly higher number of mutations compared with IDHmut-1p/19q co-deleted and IDHmut-non-1p/19q co-deleted tumours ( Fig. 1 ). Intriguingly, one tumour (2,688) was co-mutated for IDH1 (R132H) and IDH2 (P162S), but exhibited no distinguishing phenotype in terms of clinicopathology or mutation rate. 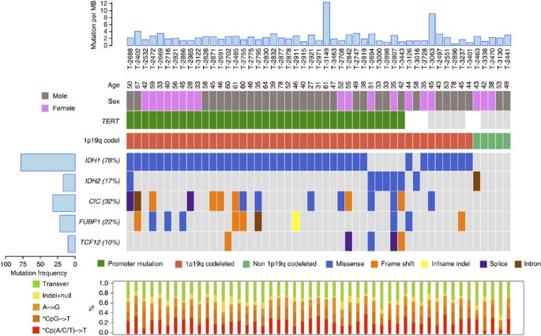Figure 1: Significantly mutated genes in anaplastic oligodendroglioma by molecular subtype. Significantly mutated genes (Q-value<0.1) identified by exome sequencing are listed byQ-value. The percentage of AO samples with mutation detected by automated calling is detailed on the left. Samples are displayed as columns, with the mutation rate plotted at the top. Samples are arranged to emphasize mutual exclusivity. Mutation types are indicated in different colours (see legend). White colour indicates no information available. Also shown is the relative proportion of base-pair substitutions within mutation categories for each tumour. Figure 1: Significantly mutated genes in anaplastic oligodendroglioma by molecular subtype. Significantly mutated genes ( Q -value<0.1) identified by exome sequencing are listed by Q -value. The percentage of AO samples with mutation detected by automated calling is detailed on the left. Samples are displayed as columns, with the mutation rate plotted at the top. Samples are arranged to emphasize mutual exclusivity. Mutation types are indicated in different colours (see legend). White colour indicates no information available. Also shown is the relative proportion of base-pair substitutions within mutation categories for each tumour. Full size image We used MutSigCV version 1.4 (ref. 8 ) to identify genes harbouring more non-synonymous mutations than expected by chance given gene size, sequence context and mutation rate of each tumour for the three molecular subtypes, respectively. As expected, we observed frequent mutations of the tumour suppressors FUBP1 (22%) located on 1p, and CIC (32%) located on 19q, which have been reported in the context of 1p/19q co-deletion ( Fig. 1 ; Supplementary Fig. 2 ); these were not mutually exclusive events ( Fig. 1 ). Also within the IDH mut-codel group, 37 of tumours tested carried TERT C228T or C250T promoter mutations (72%), none of which also carried an ATRX mutation, concordant with the previously reported finding that these are mutually exclusive events [2] . In addition to the mutation of IDH1 (78%), IDH2 (17%), CIC (32%) and FUBP1 (22%), TCF12 was also significantly mutated ( Q -value<0.1; Fig. 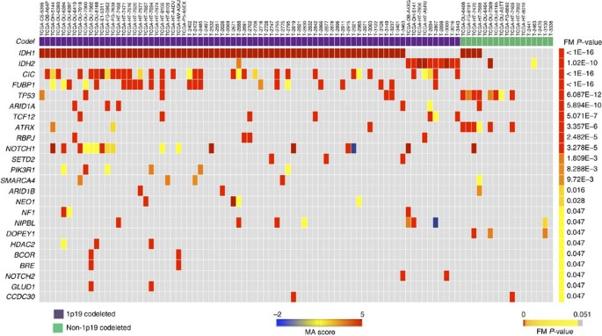Figure 2: FM-biased genes and gene modules in AO identified by Oncodrive-fm using data from this study and tumours profiled by TCGA. Heatmap shows tumours in columns and genes in rows, the colour reflecting the MutationAssessor (MA) scores of somatic mutations. FM ext. qv, correctedPvalues of the FM bias analysis using the external null distribution. 1 ; Supplementary Table 2 ). Heterozygous somatic mutations in TCF12 , which encodes the basic helix–loop–helix (bHLH) transcription factor 12 (aliases HEB , HTF4 and ALF1 ) were identified in five (1 missense, R602M; 2 splice-site, c.825+5G>T, c.1979-3_1979-delTA and 2 frameshift, E548fs*13, S682fs*14) of the 46 IDH -mutated 1p/19q co-deleted. Intriguingly, germline mutations of residues E548 and R602 have been previously shown to cause coronal craniosynostosis [10] . The availability of high-quality tumour material allowed us to generate SNP array and expression data on 31 of the cases exome sequenced. In addition to co-deletion of chromosome arms 1p/19q, we identified several other recurrent genomic alterations—mainly loses of chromosomes 4 (29%), 9p (28%) and 14q (19%); Supplementary Fig. 3 ; Supplementary Table 1 ). Notably, tumours featuring mutation of Notch-pathway genes showed significant chromosome 4 loss ( P =0.02, χ 2 -test). To identify fusion transcripts, we analysed RNA-sequencing (RNA-seq) data, which was available for 36 of the 51 tumours. After filtering, the only chimeric transcript identified was the predicted driver FGFR3–TACC3 fusion, previously described in IDH wild-type gliomas [11] , [12] , [13] , which was seen in two of the IDH wt-non-1p/19q co-deleted tumours—patients 2463 and 2441; Of note was that patient 2463 carried an IDH2 intron-5 mutation (c.679-28C>T). Incorporation of TCGA mutation data To explore the mutational spectra of AO in an independent series, we made use of data generated by The Cancer Genome Atlas (TCGA) study of low-grade glioma, which provides exome sequencing data on a further 43 AO tumours. Two of these 43 tumours harboured frameshift mutations in TCF12 (E548R and D171fs) ( Supplementary Table 2 ). As with our series, these TCF12 mutations were exclusive to IDH -1p/19q co-deleted tumours. In a combined analysis, mutations in PI3KCA , NOTCH1 and TP53 were significantly overrepresented when analysed using MutSigCV ( Q -value<0.1; Supplementary Table 2 ). In addition, mutation of ATRX and RBPJ were of borderline significance. A bias towards variants with functional impact (FM) is a feature of cancer drivers [14] . To increase our ability to identify cancer drivers and delineate associated oncogenic pathways for AO, we incorporated mutation data from multiple tumour types using Oncodrive-fm [14] implemented within the IntOGen-mutations platform [15] ( Fig. 2 ). The most recurrently mutated genes according to MutSig were also detected by Oncodrive-fm as significantly mutated ( Q -value<0.05). Oncodrive-fm also identified a number of other important mutated genes (that is, displaying high FM bias) including SETD2 , NOTCH2 , RBPJ , ARID1A , ARID1B , HDAC2 and SMARCA4 ( Fig. 2 ). Figure 2: FM-biased genes and gene modules in AO identified by Oncodrive-fm using data from this study and tumours profiled by TCGA. Heatmap shows tumours in columns and genes in rows, the colour reflecting the MutationAssessor (MA) scores of somatic mutations. FM ext. qv, corrected P values of the FM bias analysis using the external null distribution. Full size image Using all mutation results, we performed an analysis to identify pathways or gene ontologies that were significantly enriched in mutated genes. As expected, the most significantly altered pathways were linked to the tricarboxylic acid cycle and isocitrate metabolic process as a consequence of IDH mutation. Consistent with the other genes that were found significantly mutated by MutSigCV and Oncodrive-fm analysis, the Notch signalling pathway ( P =1.0 × 10 −5 , binomial test), genes involved in neuron differentiation ( P =2.0 × 10 −5 , binomial test) and genes involved in chromatin organization ( P =0.02, binomial test) were also significantly enriched for mutations ( Supplementary Data 3 ). Validation of TCF12 in an additional series of AO To identify additional TCF12 -mutated AO tumours, we conducted targeted sequencing of a further 83 AO. Five tumours harboured TCF12 mutations—G48fs*38, M260fs*5, R326S, D455fs*59 and delN606 ( Supplementary Data 1 ). On the basis of our combined sample of 134 tumours, the mutation frequency of TCF12 in AO is 7.5% (95% confidence interval 3.6–13.2%). No significant difference in patient survival in 1p/19q co-deleted AO was associated with TCF12 mutation in 69 patients ( Supplementary Fig. 4 ). While our power to demonstrate a statistically significant relationship was limited (that is, ∼ 40% for a hazard ratio of 2.0, stipulating P =0.05), we noted that patients having either TCF12 mutated or TCF12 loss of heterozygosity (LOH) tended to be associated with shorter survival ( Supplementary Fig. 4 ). To gain further insight into the role of TCF12 mutation in oligodendroglioma, we sequenced 75 grade II tumours identifying one mutation carrier (P212fs*31; Supplementary Data 1 ). The observation that the frequency of TCF12 mutations is higher in AO as compared with grade II tumours ( P =0.049, χ 2 -test) is compatible with TCF12 participating in the generation of a more aggressive phenotype. TCF12 bHLH mutants compromised transactivation To explore the functional consequences of TCF12 mutation, we tested the transcriptional activity of several mutants ( Fig. 3 ). We tested the frameshift mutations M260fs*5 and E548fs*13, which in the germline cause coronal craniosynostosis [10] and S682fs*14, since introduction of a C-terminal premature stop codon may result in escape from non-sense-mediated decay. We also tested the missense mutation R602M, which is predicted to destabilize the bHLH domain required for DNA binding and dimerization ( Fig. 3 ) and whose adjacent residue (R603) has been found recurrently mutated in colon cancer [16] . Finally, we tested the missense mutation R326S, since mutations of adjacent G327 have been reported in lung adenocarcinoma [17] . The frameshift mutants M260fs*5 and E548fs*13 completely abolished TCF12 transactivation, consistent with the lack of bHLH DNA-binding domain ( Fig. 3 ). R602M retained only 34% of WT transcriptional activity ( P =0.0018, Student’s t -test; Fig. 3 ). We did not observe significant modulation of transactivation for the R326S and S682fs*14 mutants, although the latter consistently showed decreased activity ( Fig. 3 ). 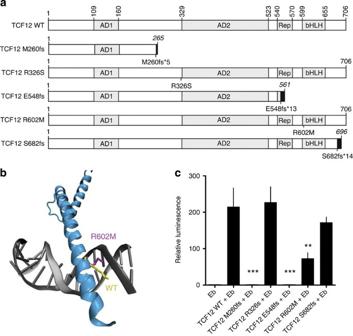Figure 3:TCF12mutations altering the bHLH domain result in impaired transactivation. (a) Schematic view of the wild-type and mutant TCF12 proteins for which the transactivation capacity has been assessed. Upper panel: wild-type human TCF12, functional domains in grey—activation domain 1 (AD1), activation domain 2 (AD2), repressor domain (Rep) and bHLH domain (bHLH). Lower panel: resulting truncated proteins. Black boxes indicate non-related amino-acid sequences resulting from frameshift mutations (fs), and truncated proteins size is in italic. (b) Schematic structure of the bHLH domain of TCF12 (blue) bound to DNA (grey). WT R602 (yellow) and mutant M602 (purple) residues are indicated. (c) E-box-luciferase reporter plasmid (Eb) was transfected alone or in combination with TCF12 wild-type or mutant expression plasmids. Both frameshift mutants that lack the bHLH DNA binding domain completely abolish TCF12 transcriptional activity. All samples were run in triplicate in four independent experiments. Data were normalized to control renilla luciferase. Values are mean±s.d. ***P=0.0002, **P=0.0018 (Student’st-test). Figure 3: TCF12 mutations altering the bHLH domain result in impaired transactivation. ( a ) Schematic view of the wild-type and mutant TCF12 proteins for which the transactivation capacity has been assessed. Upper panel: wild-type human TCF12, functional domains in grey—activation domain 1 (AD1), activation domain 2 (AD2), repressor domain (Rep) and bHLH domain (bHLH). Lower panel: resulting truncated proteins. Black boxes indicate non-related amino-acid sequences resulting from frameshift mutations (fs), and truncated proteins size is in italic. ( b ) Schematic structure of the bHLH domain of TCF12 (blue) bound to DNA (grey). WT R602 (yellow) and mutant M602 (purple) residues are indicated. ( c ) E-box-luciferase reporter plasmid (Eb) was transfected alone or in combination with TCF12 wild-type or mutant expression plasmids. Both frameshift mutants that lack the bHLH DNA binding domain completely abolish TCF12 transcriptional activity. All samples were run in triplicate in four independent experiments. Data were normalized to control renilla luciferase. Values are mean±s.d. *** P =0.0002, ** P =0.0018 (Student’s t -test). Full size image Downregulation of pathways in TCF12 bHLH mutants We profiled gene expression in 8 TCF12 -mutated and 45 wild-type tumours within 1p/19q co-deleted samples ( Supplementary Table 1 ). TCF12 mutation was associated with significant enrichment of immune response pathways ( Supplementary Data 4 ). Restricting the analysis to tumours with the TCF12 -altered bHLH domain ( n =6), we found downregulation of pathways featuring known partners of TCF12, such as TCF21, EZH2 and BMI1 (ref. 18 ) ( Supplementary Table 2 ). Interestingly, we found decreased activity of genes sets related to E-cadherin ( CDH1 ), which is a TCF12 target gene associated with tumour phenotype [18] . Since the promotor sequences of CDH1 and BMI1 feature E-box motifs and are modulated by the bHLH binding [19] , [20] , this provides a mechanistic basis for change in gene expression associated with mutant TCF12 . Mutant TCF12 proteins show subcellular localization changes We evaluated TCF12 expression and subcellular localization for all of our 11 TCF12 -mutated tumours (10 AO and 1 oligodendroglioma grade II) and 11 TCF12 wild-type tumours by immunohistochemistry. All TCF12 wild-type tumours showed nuclear expression in a heterogeneous cell population ( Fig. 4 ; Supplementary Fig. 5 ), whereas several TCF12 -mutated tumours showed nuclear and cytoplasmic staining ( Fig. 4 ; Supplementary Fig. 5 ). Interestingly, mutations abolishing transcriptional activity were associated with increased staining, suggesting inactive mutant protein accumulation. 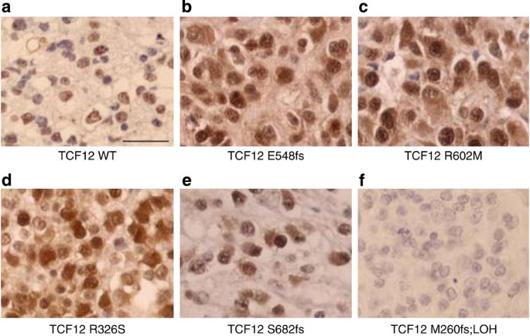Figure 4: TCF12 is highly expressed in a subset of anaplastic oligodendroglioma. Representative TCF12 immunostainings are shown: (a) wild-type TCF12 tumours show nuclear staining in a heterogeneous cell population. (b–e) Mutant TCF12 tumours show strong nuclear and cytoplasmic staining. (f) Mutant M260fs (resulting in a truncated protein) is associated with 15q21.3 LOH and shows no staining. Scale bar, 50 μm. Figure 4: TCF12 is highly expressed in a subset of anaplastic oligodendroglioma. Representative TCF12 immunostainings are shown: ( a ) wild-type TCF12 tumours show nuclear staining in a heterogeneous cell population. ( b – e ) Mutant TCF12 tumours show strong nuclear and cytoplasmic staining. ( f ) Mutant M260fs (resulting in a truncated protein) is associated with 15q21.3 LOH and shows no staining. Scale bar, 50 μm. Full size image TCF12 mutations associate with aggressive tumour phenotype We profiled the extent of necrosis, microvascular proliferation and the mitotic index available for TCF12 wild-type or mutated tumours. A significant increase in palisading necrosis ( Fig. 5 ) as well as a trend towards a higher mitotic index was associated with TCF12 mutation, consistent with a more aggressive phenotype ( Fig. 5 ). Intriguingly, tumours harbouring disruptive bHLH domain mutations exhibited the highest proportion of palisading necrosis and mitotic figures. 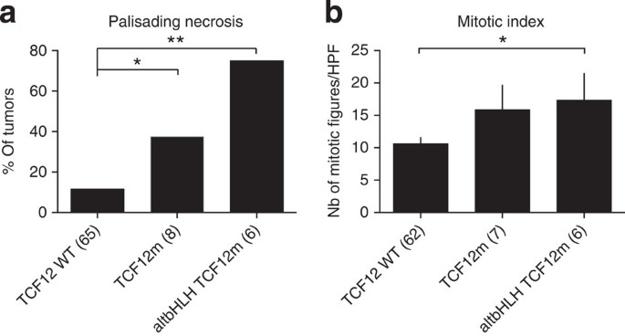Figure 5:TCF12mutation correlates with a higher necrotic and mitotic index. (a) Percentage of palisading necrosis in tumours with wild-typeTCF12, all tumours mutated forTCF12or only altered bHLHTCF12mutants; *P=0.02, **P=0.004. (b) Mitotic index inTCF12wild-type,TCF12-mutated and altered bHLHTCF12mutants; *P=0.039, mean±s.e.m. CN, copy number; LOH, loss of heterozygosity; HPF, high-power field. The number of samples is indicated in parenthesis. Figure 5: TCF12 mutation correlates with a higher necrotic and mitotic index. ( a ) Percentage of palisading necrosis in tumours with wild-type TCF12 , all tumours mutated for TCF12 or only altered bHLH TCF12 mutants; * P =0.02, ** P =0.004. ( b ) Mitotic index in TCF12 wild-type, TCF12 -mutated and altered bHLH TCF12 mutants; * P =0.039, mean±s.e.m. CN, copy number; LOH, loss of heterozygosity; HPF, high-power field. The number of samples is indicated in parenthesis. Full size image Our genome sequencing of AO has confirmed the mutually exclusive mutational profile in IDH mut-1p/19q co-deleted and IDH mut non-1p/19q co-deleted tumour subtypes, which reflect distinct molecular mechanisms of oncogenesis—consistent with the requirement for either 1p/19q co-deletion or TP53 mutation post IDH mutation. Moreover, as previously proposed, the genomic abnormalities in IDH mut-1p/19p co-deleted tumours are consistent with one common mechanism of tumour initiation being through 1p/19q loss, mutation of IDH1 or IDH2 and TERT activation through promoter mutation [2] , which in turn predisposes to deactivation of CIC , FUBP1 , NOTCH and activating mutations/amplifications in the PI3K pathway. We identified and replicated mutations in TCF12 , a bHLH transcription factor that mediates transcription by forming homo- or heterodimers with other bHLH transcription factors. Tcf12 is highly expressed in neural progenitor cells during neural development [21] and in cells of the oligodendrocyte lineage [22] . We found that mutations generating truncated TCF12 lacking the bHLH DNA-binding domain abrogate the transcriptional activity of TCF12. In addition, single residue substitutions such as R602M within the bHLH domain also dramatically reduce TCF12 transcriptional ability. Finally, we found that the loss of TCF12 transcriptional activity was associated with a more aggressive tumour phenotype. Although speculative, our expression data provides evidence that the effects of TCF12 mutation on AO development may be mediated in part through E-cadherin related pathway. Indeed, this was one of the pathways down-regulated in mutated tumours and intriguingly CDH1 has been implicated in metastatic behaviour in a number of cancers [18] , [23] . It is likely that some TCF12 mutations may have subtle effects on bHLH function or act through independent pathways. Irrespective of the downstream effects of TCF12 mutation on glioma, our data are compatible with TCF12 having haploinsufficient tumour suppressor function. TCF12 haploinsufficiency has previously been reported in patients with coronal craniosynostosis and in their unaffected relatives [10] . Strikingly, 3 of the 11 mutations we identified in AO, which concern residues M260, E548 and R602, cause coronal craniosynostosis [10] , [24] . Although speculative, collectively these data raise the possibility that carriers of germline TCF12 mutations may be at an increased risk of developing AO. To our knowledge, this study represents the largest sequencing study of AO conducted to date. However, given the number of tumour-normal pairs we have analysed and the mutational frequency in AO, we were only well powered to identify genes that have a high-frequency mutations (that is, >10%). Hence further insights into the biology of AO should be forthcoming through additional sequencing initiatives and meta-analyses of these data. Patient samples and consent Samples were obtained with informed and written consent and the study was approved by Comité de Protection des Personnes Ile de France-VI (October 2008) of respective hospitals participating in the Prise en charge des oligodendrogliomes anaplasiques (POLA) network. All patients were aged 18 years or older at diagnosis, and tumour histology was centrally reviewed and validated according to World Health Organization (WHO) guidelines [25] . Exome sequencing was conducted on samples from 51 AO patients (33 male; median age 49 years at diagnosis, range 27–81). For targeted follow-up analyses, we studied the tumours from an additional 83 AO patients and 75 patients with grade II tumours. A summary of each of the tumour cohorts and respective pathological information on the patients is provided in Supplementary Table 1 . DNA and RNA extraction Germline DNA was extracted from EDTA-venous blood samples using QIAquick PCR Purification Kits (Qiagen Ltd). Tumour DNA was extracted from snap-frozen tumour samples using the iPrep ChargeSwitchH Forensic Kit, according to manufacturer’s recommendations. DNAs were quantified and qualified using a NanoVue Plus spectrophotometer (GE Healthcare Life Sciences) and gel electrophoresis. RNA was extracted from tumours lysed by Lysing Matrix D tube and FastPrep instrument (MP Biomedicals) using the iPrep Trizol Plus RNA Kit (Life Technologies). Stringent criteria for RNA quality were applied to rule out degradation, specifically a 28S/18S ratio >1.8. SNP array analysis In total, 115 samples from tumours were genotyped using Illumina SNP microarrays: 32 samples with Illumina 370-Duo 1.0 BeadChips, 31 with Human610-Quad, 46 with HumanOmniexpress-12V1 and 6 with HumanCore-12v1. Raw fluorescent signals were imported into BeadStudio software (Illumina) and normalized to obtain log R ratio and B-allele frequency (BAF) values. The tQN normalization procedure was then applied to correct for asymmetry in BAF signals due to bias between the two dyes used in Illumina assays. Genomic profiles were divided into homogeneous segments by applying the circular binary segmentation algorithm to both log R ratio and BAF values. We then used the Genome Alteration Print method to determine the ploidy of each sample, the level of contamination with normal cells and the allele-specific copy number of each segment. Chromosome aberrations were defined using empirically determined thresholds as follows: gain, copy number ≥ploidy+1; loss, copy number ≤ploidy −1; high-level amplification, copy number >ploidy+2; homozygous deletion, copy number=0. Finally, we considered a segment to have undergone LOH when the copy number of the minor allele was equal to 0. Lists of homozygous deletions and focal amplifications, defined by at least five consecutive probes, were generated and verified manually to remove doubtful events. Significantly recurrent copy number changes were identified using the GISTIC2.0 algorithm [26] . TERT promoter mutation sequencing Characterized mutations in the TERT promoter, C228T and C250T variants with G>A nucleotide substitutions at genomic positions 1,295,228 bp and 1,295,250 bp (hg19), respectively, were obtained by Sanger sequencing. Primer sequences were: TERT-F—5′-GGCCGATTCGACCTCTCT-3′ and TERT-R 5′-AGCACCTCGCGGTAGTGG-3′. Whole-exome sequencing DNA was quantified using the Quant-iT PicoGreen dsDNA Assay Kit (Life Technologies). Libraries were generated robotically using the SureSelectXT Automated Human All Exon Target Enrichment for Illumina Paired-End Multiplexed Sequencing (Agilent) as per the manufacturer’s recommendations. Libraries were quantified using the Quant-iT PicoGreen dsDNA Assay Kit (Life Technologies) and the Kapa Illumina GA with Revised Primers-SYBR Fast Universal kit (D-Mark). Average size of the fragment was determined using a LaChip GX (PerkinElmer) instrument. Sequencing was performed by pooling four libraries per lane at a 9-pM dilution on an Illumina HiSeq 2,000 instrument for 2 × 100 cycles using the recommended manufacturer’s conditions. PhiX control was added at 1% on each lane. BCL2FASTQ (Illumina) was used to convert bcl files to fastqs (v 1.8.4). Coverage statistics are summarized in Supplementary Fig. 1 . Paired-end fastq files were extracted using Illumina CASAVA software (v.1.8.1, Illumina) and aligned to build 37 (hg19) of the human reference genome using Stampy and Burrows–Wheeler Aligner [27] , and PCR duplicates were removed with PicardTools 1.5. We assessed coverage of consensus coding sequence bases using Genome Analysis Toolkit [28] v2.4-9. Somatic single-nucleotide variants were called using MuTect [29] and the Genome Analysis Toolkit v2.4-9, and indels using IndelGenotyper. We excluded potential Covaris-induced mutations as per Costello et al . [30] using in-house scripts. Confirmation of selected single-nucleotide variants including TCF12 , CIC , FUBP1 , SYNE1 , FAT1 , SETD2 , RBPJ , NOTCH1 , IDH1 and IDH2 was performed by Sanger sequencing implemented on ABI 3,300 × l platforms (Applied Biosystems, Foster City, USA). Primer sequences are detailed in Supplementary Data 5 . In all cases, Sanger sequencing was 100% concordant with next-generation sequencing. We used MutSigCV [8] version 1.4 to identify genes harbouring more non-synonymous mutations than expected by chance, given gene size, sequence context and the mutation rate. We used as genomic covariates the mean expression level of each gene in our AO expression data set, the DNA replication time and the HiC statistic of chromatin state available in MutSig reference files. To increase our ability to identify cancer drivers and delineate associated oncogenic pathways for AO, we incorporated mutation data from multiple tumour types using Oncodrive-fm [14] implemented within the IntOGen-mutations platform [15] . Transcriptome sequencing Extracted RNA was cleaned using the RNeasy MinElute Cleanup Kit (Qiagen) and the RNA integrity assessed using an Agilent 2,100 Bioanalyzer and quantified using a Nanodrop 1,000. Libraries for stranded total RNA-seq were prepared using the Illumina Stranded Total RNA protocol (RS-122-2301). Libraries were assessed by the Agilent 2,100 Bioanalyzer. Sequencing was performed by pooling four libraries per lane at a 9-pM dilution on an Illumina HiSeq 2,000 instrument for 2 × 100 cycles using the recommended manufacturer’s conditions. PhiX control was added at 1% on each lane. BCL2FASTQ was used to convert bcl files to fastqs (v 1.8.4). Paired-end reads from RNA-seq were aligned to the following database files using Burrows–Wheeler Aligner 0.5.5: (i) the human GRCh37-lite reference sequence, (ii) RefSeq, (iii) a sequence file representing all possible combinations of non-sequential pairs in RefSeq exons and (iv) the AceView database flat file downloaded from UCSC, representing transcripts constructed from human expressed sequence tag (ESTs). The mapping results from databases (ii)-(iv) were aligned to human reference genome coordinates. The final BAM file was constructed by selecting the best alignment. To identify fusion transcripts, we analysed RNA-seq data using Chimerascan software [31] (version 0.4.5). As advocated, algorithmic output was analysed for high-confidence fusion transcripts imposing filters: (i) spanning reads >2 (ii) total supported reads ≥10 (ref. 32 ). In absence of corresponding paired normal tissue samples, we made use of data from the human body map project data to identify fusions seen in normal tissue. TCF12 sequencing in the validation series PCR amplification of 21 amplicons covering each exon of TCF12 on DNA extracted from fresh-frozen tumours were performed using Fluidigm technology according to the manufacturer’s recommendations. The 21 PCR products from one tumour sample were then equimolarly pooled and submitted to the MiSeq (Illumina) sequencing as per the manufacturer’s protocol. All mutations were validated by Sanger sequencing. Somatic mutations were confirmed using paired constitutional DNA. mRNA expression profiling Gene expression profiles of 71 samples were analysed using Affymetrix Human Genome U133 Plus 2.0 arrays. All samples were normalized in batches using the RMA algorithm (Bioconductor affy package), and probe set intensities were then averaged per gene symbol. Identification of significantly mutated pathways Gene set member lists were retrieved online from MSigDB [33] , GO [34] and SMD [35] databases. We searched for gene sets harbouring more damaging mutations than expected by chance. Given the set G of all the genes sequenced with sufficient coverage, the set S of tumour samples (of size n ) and any gene set P, we calculated the probability of observing a number of mutations equal or greater to that observed in P across the n samples according to a binomial law B ( k , p ), with k = n × L (P) and the mutation rate p = A (G, S)/( n × L ( G )), where L (X) is the sum of the lengths (in bp) of all genes/exons from a gene set X, and A (G, S) is the total number of mutations observed in all the targeted sequences across all the samples from S. Deregulated gene sets in TCF12 mutant samples We performed a moderate t -test using LIMMA R package to identify significantly differentially expressed genes between TCF12 mutant samples and TCF12 wild-type samples ( P <0.05 and absolute log fold change >0.6). Biological pathways and gene set member lists were retrieved online from MSigDB [33] , GO [34] and SMD [35] databases. Enrichment P values were computed from a hypergeometric test between those gene sets and the initial list of differentially expressed genes. To visualize gene set activity, for each gene set defined as target genes of either CDH1 , TCF21 , BMI1 , EZH2 and found to be significantly deregulated in TCF12 bHLH-altered samples compared with TCF12 wild-type samples in O3 samples with co-deletion, we retrieved the complete member list from MSigDB [33] and computed a global mean gene expression value in each sample. We then ranked the samples according to the later global mean expression value for each of these gene sets. Structure modelling The Swiss Model [36] server was used to model mutated TCF12 and VMD software [37] used to align the structures of wild-type and mutated TCF12 proteins with STAMP (STructural Alignment of Multiple Proteins) [38] . Prediction of the functional effect of the R602M mutation on TCF12 was made using Project HOPE [39] . Statistical analysis Statistical analysis was carried out using R3.0.1 software. A P value ≤0.05 was considered to be significant. Continuous variables were analysed using the Student’s t -test or Mann–Whitney test. Categorical data were compared using Fisher’s exact test or the χ 2 -test. Overall survival of patients was the end point of the analysis. Survival time was calculated from the date of tumour diagnosis to the date of death. Patients who were not deceased were censored at the date of last contact. Mean follow-up time was computed among censored observations only. Kaplan–Meier survival curves according to genotype were generated and the homogeneity of the survival curves between genotypes was evaluated using the log-rank test. Power to demonstrate a relationship between mutation status and overall survival was estimated using sample size formulae for comparative binomial trials [40] . Cell culture Human embryonic kidney HEK293T cell line (American Type Culture Collection) was maintained in a 5% CO 2 -regulated incubator in DMEM Glutamax (Life Technologies), completed with 10% fetal bovine serum and penicillin/streptomycin (Life Technologies). Plasmid construction To construct the TCF12 wild-type plasmid, we cloned, by Gateway recombination (Life Technologies), a pENTR221 TCF12 Ultimate ORF Clone (Life Technologies) into a pDEST12 lentiviral vector (kind gift from P. Ravassard), under the control of hCMV promoter. The M260fs*5 and R326S mutations were generated by PCR mutagenesis using the Q5 Site-directed Mutagenesis kit (New England Biolabs) on pENTR221 TCF12 plasmid (primer sequences are detailed in Supplementary Data 5 ) and then cloned into the pDEST12 vector by LR Gateway cloning. Synthetic NdeI/MfeI fragments (encompassing sequences from exon 16 to the TAG stop codon of the ENST00000438423 isoform), containing the mutations E548fs*13, R602M and S683fs*14, were obtained from GeneCust, then substituted into pENTR221 and finally cloned by Gateway recombination into the pDEST12 plasmid. All expression plasmids were sequenced before use. Luciferase expression assays For each experiment, 10 5 exponentially growing HEK293T cells were seeded in 12-well plates and transfected 24 h later using Fugene6 (Promega), according to manufacturer’s instructions, with 0.3 μg of a reporter plasmid encoding firefly luciferase under the control of an E-box-responsive element (Eb, kind gift from A. Lasorella), or 0.3 μg of Eb plasmid and 0.7 μg of a TCF12 wild-type expression plasmid, or 0.3 μg of Eb plasmid and 0.7 μg of either TCF12 mutant (M260fs*5, R326S, E548fs*13, R602M or S628fs*14) expression plasmid. For all points, data were normalized by adding 30 ng of renilla luciferase expression plasmid (pGL4.73, Promega, gift from F. Toledo). Cells were harvested 24 h after transfection, and luminescence was monitored using the Dual-Glo Luciferase assay system (Promega), according to the manufacturer’s instructions, on a Spectramax M4 instrument and SoftMax Pro 6.2.2 software. All samples were run in triplicate, in four independent experiments. Immunohistochemistry Paraffin-embedded tumour sections were deparaffinized using standard protocols. Heat-mediated antigen retrieval was achieved by boiling sections in a pressure cooker with Citrate buffer at pH 6. Sections were blocked in 10% goat serum in PBS+0.5% Triton X-100 for 30 min prior to incubation with an anti-TCF12 antibody (Proteintech Cat no. : 14419-1-AP) and then revealed using the Polink-2 HRP Plus Rabbit DAB Detection System (GBI Labs:D39-6). Photographs were taken at × 400 magnification and processed using AxioVision software (Zeiss). The mitotic index in tumours was recorded as the number of mitotic figures in 10 high-power fields. TCGA data To complement our analysis, we made use of exome sequencing data on AO tumours generated by the TCGA ( Supplementary Data 2 ). Accession codes: All whole-exome sequencing and transcriptome data have been deposited at the European Genome-phenome Archive (EGA), which is hosted by the European Bioinformatics Institute (EBI), under the accession code EGAS00001001209. mRNA expression and SNP data can be accessed through ArrayExpress under accession numbers E-MTAB-2768 for mRNA expression data, and E-MTAB-3457 , E-MTAB-3458 , E-MTAB-2772 and E-MTAB-2771 for SNP data. How to cite this article: Labreche, K. et al . TCF12 is mutated in anaplastic oligodendroglioma. Nat. Commun. 6:7207 doi: 10.1038/ncomms8207 (2015).